Shh-mediated degradation of Hhip allows cell autonomous and non-cell autonomous Shh signalling The distribution of Sonic Hedgehog (Shh) is a highly regulated and critical process for development. Several negative feedback mechanisms are in place, including the Shh-induced upregulation of Hedgehog-interacting protein (Hhip). Hhip sequesters Shh, leading to a non-cell autonomous inhibition of the pathway. Hhip overexpression has a severe effect on neural tube development, raising the question why normal sites of Hhip expression have a seemingly unimpaired response to Shh. Here we show that although Hhip is able to leave its sites of synthesis to inhibit Shh non-cell autonomously, activation of Smoothened (Smo) drastically increases Hhip internalization and degradation cell autonomously. Although Hhip is unable to cell autonomously inhibit the consequences of Smo activation, it can inhibit the Shh response non-cell autonomously. Our data provide a mechanism by which the Shh ligand can activate the response and negate cell autonomous effects of Hhip, while Hhip can still induce non-cell autonomous inhibition. Signal transduction by members of the Hedgehog (Hh) family of molecules is essential during development. As morphogens, Hh proteins are secreted from localized sources to induce distinct concentration-dependent cellular responses. Highly regulated feedback mechanisms are in place to ensure that Hh gradients are established appropriately within responding tissues. Of all the Hh ligands, Sonic Hedgehog (Shh) has been most intensely studied, for instance in neural tube patterning. Shh is synthesized in the notochord and in the floor plate of the developing neural tube, providing sources of a ventral to dorsal gradient. This Shh gradient induces a spatially and temporally dependent expression of transcription factors that determine specific neural cell fates. The Shh response is initiated by two membrane proteins, Patched1 (Ptch1) and Smoothened (Smo). Ptch1 is the receptor for Hh, whereas Smo is the activator of the downstream pathway. In the absence of Hh ligands, Ptch1 suppresses the activity of Smo, which is released upon Hh binding to Ptch1, allowing Smo to activate its downstream targets [1] . Shh gradient formation is regulated by several cell surface proteins that bind to and limit the distribution of Shh. One of these proteins is Hedgehog-interacting protein (Hhip), a vertebrate-specific protein that binds to Shh [2] . Like Ptch1 , Hhip is transcriptionally upregulated in response to Shh signalling and consequently Hhip is highly expressed just dorsal to the floor plate. Hhip overexpression in animals causes severe skeletal and pituitary defects [2] , [3] , whereas Hhip loss of function causes an increase in Hh signalling resulting in lung, skeleton, gut and pancreas malformations [4] , [5] . Interestingly, the consequences of Hhip loss of function are relatively minor in the spinal cord, although the function of Hhip in the developing spinal cord becomes apparent when Ptch1 activity is reduced [6] , [7] . From these studies, the general idea has emerged that Hhip acts at the cell surface of the cell that expresses it to bind and sequester Shh, making it unavailable to Ptch1 for pathway activation both cell autonomously and to nearby cells. This sequestration model is consistent with the proposed role of Hhip function as a barrier that decreases the amount of Shh available to cells distal to the Shh source and Hhip expression domain, resulting in the inhibition of Shh activity non-cell autonomously. In the brain, soluble forms of Hhip have been detected [8] , raising questions regarding the nature of the non-cell autonomous inhibition by Hhip. Here we investigated the distinct cell autonomous and non-cell autonomous roles of Hhip in the inhibition of the Shh response. Consistent with other reports [6] , [9] , we show that Hhip expression by itself had a severe effect on neural tube development, raising the question of why the Shh-induced expression of Hhip does not result in a cell-autonomous inhibition of the Shh response. We identify a mechanism by which activation of Smo results in a rapid internalization and degradation of Hhip, thus mitigating the consequences of Hhip expression cell autonomously, but allowing Hhip to inhibit the Shh response at a distance. Shh-binding domain of Hhip is necessary for Shh inhibition Hhip is a multidomain protein. To assess the functions of these domains, we created the following deletions of: the Shh-binding domain, HhipΔL2 (ref. 10 ); the two epidermal growth factor (EGF) domains, HhipΔEGF, and a stretch of 20 amino acids that contains 9 arginines, which we called as the arginine-rich region (AR), HhipΔAR ( Fig. 1a ). The AR is located within the cysteine-rich domain (CRD) of Hhip, which shares characteristics with Frizzled-like CRDs [10] , [11] . The mutants were assessed for their ability to inhibit the Shh response in the developing chick neural tube. At high concentrations, Shh induces motor neuron precursors, which upon becoming postmitotic, express the marker Hb9 (ref. 12 ). Even at low concentrations, Shh represses Pax7 expression, limiting Pax7 to the dorsal half of the neural tube [13] . We examined the expression of these markers as a measure of Shh activity in the neural tube. 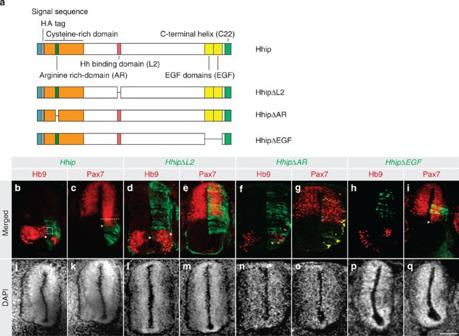Figure 1: The Hedgehog-binding domain is required for the inhibition of the Shh response by Hhip. (a) Schematic diagram of the Hhip protein domains, and deletion mutants generated. (b–q) Cross-sections of chick neural tubes electroporated at stage 10 Hamburger Hamilton (HH) and analysed at stages 18–20 are shown. ElectroporatedpMES-Hhip(b,c,j,k),pMES-HA-HhipΔL2(d,e,l,m),pMES-HA-HhipΔAR(f,g,n,o) andpMES-HA-HhipΔEGF(h,i,p,q) is shown in green. Sections were stained with anti-Hb9 (b,d,fandh) or anti-Pax7 (c,e,gandi) antibodies, labelled in red. Cells expressing wild-type Hhip inhibit Hb9 expression in those cells (denoted by the dashed square box,b). Hhip also inhibits Hb9 expression in neighbouring cells (denoted by the arrowhead,b). In addition, wild-type Hhip cell autonomously induced Pax7 expression (denoted by yellow arrowhead, panelc) and non-cell autonomously (dorsal to the dashed line,c). (d) Arrowheads indicate co-expression of HhipΔL2 and Hb9 in the same cells. Below the merged images are the corresponding 4,6-diamidino-2-phenylindole (DAPI) nuclei stains (j–q). Fisher’s exact test shows that the effects of HhipP<0.0001 (n=10), HhipΔARP<0.0001 (n=11) and HhipΔEGFP=0.0152 (n=6) are significant. HhipΔLp2 has no effect;P=1 (n=10). Scale bar, 50 μm (q). Figure 1: The Hedgehog-binding domain is required for the inhibition of the Shh response by Hhip. ( a ) Schematic diagram of the Hhip protein domains, and deletion mutants generated. ( b – q ) Cross-sections of chick neural tubes electroporated at stage 10 Hamburger Hamilton (HH) and analysed at stages 18–20 are shown. Electroporated pMES-Hhip ( b , c , j , k ), pMES-HA-HhipΔL2 ( d , e , l , m ), pMES-HA-HhipΔAR ( f , g , n , o ) and pMES-HA-HhipΔEGF ( h , i , p , q ) is shown in green. Sections were stained with anti-Hb9 ( b , d , f and h ) or anti-Pax7 ( c , e , g and i ) antibodies, labelled in red. Cells expressing wild-type Hhip inhibit Hb9 expression in those cells (denoted by the dashed square box, b ). Hhip also inhibits Hb9 expression in neighbouring cells (denoted by the arrowhead, b ). In addition, wild-type Hhip cell autonomously induced Pax7 expression (denoted by yellow arrowhead, panel c ) and non-cell autonomously (dorsal to the dashed line, c ). ( d ) Arrowheads indicate co-expression of HhipΔL2 and Hb9 in the same cells. Below the merged images are the corresponding 4,6-diamidino-2-phenylindole (DAPI) nuclei stains ( j – q ). Fisher’s exact test shows that the effects of Hhip P <0.0001 ( n =10), HhipΔAR P <0.0001 ( n =11) and HhipΔEGF P =0.0152 ( n =6) are significant. HhipΔLp2 has no effect; P =1 ( n =10). Scale bar, 50 μm ( q ). Full size image Ectopic expression of Hhip in the ventral neural tube resulted in Hb9 inhibition ( Fig. 1b ) and an expansion of the Pax7 domain ( Fig. 1c ), demonstrating an inhibition of the Shh response. The expansion of Pax7 included expression in cells that did not express Hhip, indicating that Hhip inhibited the Shh response in neighbouring cells. These findings are in agreement with previous observations that demonstrate a non-cell autonomous action of Hhip on Shh in the neural tube [6] , [9] . Expression of HhipΔL2 did not inhibit Shh activity as both Hb9 and Pax7 expression were not affected ( Fig. 1d,e ), confirming that the Shh-binding function of Hhip is necessary to inhibit the Shh response in the neural tube and is in line with previous experiments in zebrafish and cell culture [10] , [14] . Moreover, HhipΔAR and HhipΔEGF inhibited the Shh response similar to wild-type Hhip ( Fig. 1f–i ), indicating that these domains are dispensable for Hhip inhibition of Shh. HhipΔEGF-mediated Hb9 inhibition and Pax7 expansion included domains ventral to the HhipΔEGF-expressing cells ( Fig. 1h,i ). Currently, Hhip is thought to act at the cell surface of the cell that expresses it (cell autonomously), binding and sequestering Shh, making it unavailable to Ptch1 for pathway activation in neighbouring cells. This model implies that the main effects of Hhip are a barrier or a sieve that slows down Shh transport, resulting in inhibition of Shh activity non-cell autonomously. If Hhip indeed acts as a barrier, then Hhip expression must be between the Shh source and the domain where the Shh response is inhibited. Our results are inconsistent with such a barrier function of Hhip, and a possible explanation for this is the existence of a form of Hhip that is released from cells and moves into the Shh gradient to inhibit the Shh response at a distance. Hhip released from cells interacts with and inhibits Shh In electroporated neural tubes, the side of the neural tube expressing Hhip was often smaller than the opposite side ( Fig. 1j–q ), consistent with an important function of Shh as a mitogen and the interference by Hhip with this role [15] . To determine whether Hhip is released from cells that synthesize it, or if the observation in vivo was due to the effect of a deformed/shortened neural tube, we assessed the localization of Hhip in cultured cells. Madin–Darby canine kidney cells transfected with Hhip , or an untethered form of Hhip lacking the C-terminal membrane anchor, HhipΔC22 , in combination with GFP , were co-cultured with (independently) Shh -transfected cells. Both Hhip and HhipΔC22 were detected on Shh-expressing cells, but not on other cells ( Fig. 2d,f ), likely due to a direct interaction between Hhip and Shh. These observations support the idea that Hhip is released from cells that synthesize it, indicating that at least some of the non-cell autonomous Shh inhibition is due to Hhip release. 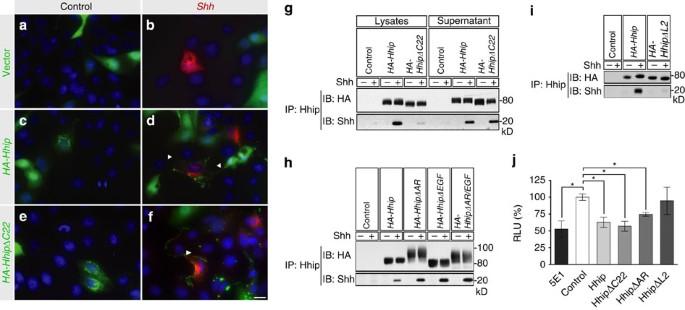Figure 2: Hhip is released from cells and binds to Shh to inhibit the Shh response. (a–f) Madin–Darby canine kidney (MDCK) cells co-transfected withpcDNA-HA-HhipandpcDNA-GFP(cytoplasmic green) and co-cultured with cells independently transfected withpRK5-Shhor an empty vector control were stained with anti-HA, antibody shown as green puncta, anti-Shh antibody (red) and 4,6-diamidino-2-phenylindole (DAPI; blue). Arrowheads point to Hhip puncta. Scale bar, 20 μm (f). HEK293T cells were transfected separately, then co-cultured for 24 h and lysed. Co-immunoprecipitation of Hhip mutants and Shh from cell lysates (g,i) and from cell culture medium (g,h). (g) Shh was co-immunoprecipitated with wild-type Hhip and soluble HhipΔC22 from both cell lysates and cell culture supernatants. (h) HhipΔAR, HhipΔEGF and Hhip ΔAR/EGF bind to Shh. (i) HhipΔL2 mutant does not co-immunoprecipitate with Shh. (j) Shh-LIGHT II cells were co-cultured with MIA PaCa-2 cells, and after incubation with 5E1 blocking antibody or Hhip conditioned medium, cells were lysed and luciferase activity was measured. RLU; relative light units,n=3±s.e.m., *P<0.008 using Student’st-test. Figure 2: Hhip is released from cells and binds to Shh to inhibit the Shh response. ( a – f ) Madin–Darby canine kidney (MDCK) cells co-transfected with pcDNA-HA-Hhip and pcDNA-GFP (cytoplasmic green) and co-cultured with cells independently transfected with pRK5-Shh or an empty vector control were stained with anti-HA, antibody shown as green puncta, anti-Shh antibody (red) and 4,6-diamidino-2-phenylindole (DAPI; blue). Arrowheads point to Hhip puncta. Scale bar, 20 μm ( f ). HEK293T cells were transfected separately, then co-cultured for 24 h and lysed. Co-immunoprecipitation of Hhip mutants and Shh from cell lysates ( g , i ) and from cell culture medium ( g , h ). ( g ) Shh was co-immunoprecipitated with wild-type Hhip and soluble HhipΔC22 from both cell lysates and cell culture supernatants. ( h ) HhipΔAR, HhipΔEGF and Hhip ΔAR/EGF bind to Shh. ( i ) HhipΔL2 mutant does not co-immunoprecipitate with Shh. ( j ) Shh-LIGHT II cells were co-cultured with MIA PaCa-2 cells, and after incubation with 5E1 blocking antibody or Hhip conditioned medium, cells were lysed and luciferase activity was measured. RLU; relative light units, n =3±s.e.m., * P <0.008 using Student’s t -test. Full size image Previous studies have mapped the Hhip- and Shh-binding regions important for interaction and have also noted that lipid modification of Shh is not a requirement [2] , [10] , [11] . However, we wanted to assess the interaction between Shh and the Hhip protein that is released from cells. Cells expressing either Hhip or Shh were co-cultured, and Hhip and Shh were co-immunoprecipitated from cell lysates and culture medium. Hhip bound to Shh in both cell lysates and medium ( Fig. 2g ). In contrast, the untethered mutant, HhipΔC22, showed robust binding in culture medium but very little in cell lysates, indicating that most was released from cells. Both HhipΔEGF and HhipΔAR were able to bind to Shh in both lysates (data not shown) and culture medium ( Fig. 2h ), indicating that the AR and EGF domains do not play a role in the release of Shh from cells or binding to Shh. HhipΔL2 did not bind to Shh ( Fig. 2i ). These data indicate that wild-type Hhip, despite having a C-terminal helix inserted into the membrane, is released from cells and able to bind to Shh via Hhip L2 domain. To assess whether released Hhip can inhibit signalling by endogenously expressed Shh, we performed reporter assays in Shh-LIGHT II cells [16] that were cultured in aggregate with MIA PaCa-2 cells, which express high amounts of Shh ligand [17] . MIA PaCa-2-induced Gli-luciferase activity was Shh ligand-mediated; addition of the Shh-blocking antibody 5E1 decreased pathway activity ( Fig. 2j ). Hhip, HhipΔC22 and HhipΔAR in conditioned medium all significantly reduced Gli-luciferase activity, further supporting the efficacy of a non-cell autonomous action of Hhip. Shh and Smo induce Hhip degradation cell autonomously Hhip was detectable when co-cultured with cells that were independently transfected with Shh ( Fig. 2d ), but we were unable to detect Hhip in cells that also expressed Shh. Although Hhip and Shh are not known to be expressed in the same cells in vivo , we nevertheless decided to examine why Shh expression in the same cells prevented the detection of Hhip. HEK 293T cells were co-transfected with Hhip and Shh or the inactive C-terminal processed form of Shh, ShhC ( Fig. 3a , lanes 1 and 2). Hhip was present at much lower levels in cells expressing Shh than in cells expressing ShhC. This effect was not a consequence of vector backbone differences ( Fig. 3b , lanes 19–21), and Shh was not affected by Hhip co-transfection ( Fig. 3b , lanes 3 and 6). To further test whether Shh/Hhip binding is important for the loss of Hhip, we co-transfected HhipΔL2 with Shh or ShhC (lanes 11 and 12) and found that Shh also caused a loss of HhipΔL2. These results indicate that Hhip stability is independent of Hhip binding to Shh and instead implicates Shh pathway activation in the degradation of Hhip. 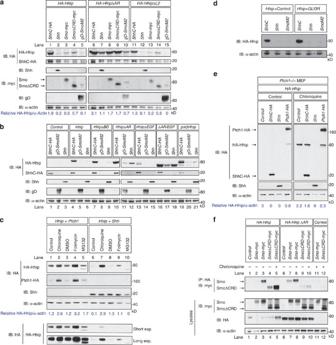Figure 3: Shh and Smo increase Hhip protein turnover. (a) HEK293T cells were transiently co-transfected withHA-Hhip(lanes 1–5),HA-HhipΔAR(lanes 6–10) andHA-HhipΔL2(lanes 11–15) and the indicated Shh or Smo constructs. Western blot of whole-cell lysates were immunoblotted with the indicated antibodies. (b) HEK293T cells were co-transfected with Hhip mutants andShhC-HA,gD-SmoM2 orShh. Western blot analyses of whole-cell lysates were immunoblotted with the indicated antibodies. Co-transfection ofprk5-HA-Hhipandprk5-Shh(lanes 19 and 20) resulted in the same result aspcDNA3-HA-Hhipandprk5-Shh. In addition, the Hhip AR region is involved in Hhip stability (lanes 10–12, 16–18). (c) HEK293T cells were transiently co-transfected withHA-HhipandPtch1-HAorShh. After 24 h post-transfection, cells were treated with water (control), 100 μM chloroquine, dimethylsulphoxide, 100 nM folimycin A or 5 μM MG132 for an additional 24 h before lysis. For the Hhip HA immnunoblot, lanes 1–5 represent a shorter exposure than lanes 6–10, the entire blot of both exposures is below. (d) As forc, cells were co-transfected with control vector orGLI3R. (e)Ptch1−/−MEFs were co-transfected withHA-Hhipand indicated constructs, and 24 h after transfection, cells were treated with 100 μM chloroquine for 4 h. (f) HEK293T cells were transiently co-transfected withHA-Hhip(lanes 1–5),HA-HhipΔAR(lanes 6–10) or empty vector control (lanes 11 and 12) and either empty vector control,Smo-mycorSmoΔCRD-mycand treated with 100 μM chloroquine. Cell lysates were immunoprecipitated with anti-HA antibody and immunoblotted with anti-Myc antibody. Figure 3: Shh and Smo increase Hhip protein turnover. ( a ) HEK293T cells were transiently co-transfected with HA-Hhip (lanes 1–5), HA-HhipΔAR (lanes 6–10) and HA-HhipΔL2 (lanes 11–15) and the indicated Shh or Smo constructs. Western blot of whole-cell lysates were immunoblotted with the indicated antibodies. ( b ) HEK293T cells were co-transfected with Hhip mutants and ShhC-HA , gD -SmoM2 or Shh . Western blot analyses of whole-cell lysates were immunoblotted with the indicated antibodies. Co-transfection of prk5-HA-Hhip and prk5-Shh (lanes 19 and 20) resulted in the same result as pcDNA3-HA-Hhip and prk5-Shh . In addition, the Hhip AR region is involved in Hhip stability (lanes 10–12, 16–18). ( c ) HEK293T cells were transiently co-transfected with HA-Hhip and Ptch1-HA or Shh . After 24 h post-transfection, cells were treated with water (control), 100 μM chloroquine, dimethylsulphoxide, 100 nM folimycin A or 5 μM MG132 for an additional 24 h before lysis. For the Hhip HA immnunoblot, lanes 1–5 represent a shorter exposure than lanes 6–10, the entire blot of both exposures is below. ( d ) As for c , cells were co-transfected with control vector or GLI3R . ( e ) Ptch1 −/− MEFs were co-transfected with HA-Hhip and indicated constructs, and 24 h after transfection, cells were treated with 100 μM chloroquine for 4 h. ( f ) HEK293T cells were transiently co-transfected with HA-Hhip (lanes 1–5), HA-HhipΔAR (lanes 6–10) or empty vector control (lanes 11 and 12) and either empty vector control, Smo-myc or SmoΔCRD-myc and treated with 100 μM chloroquine. Cell lysates were immunoprecipitated with anti-HA antibody and immunoblotted with anti-Myc antibody. Full size image To test whether Hhip degradation is mediated by the activation of the pathway, we co-transfected Hhip with wild-type Smo, or an activated form of Smo, SMOM2 (ref. 18 ). Both Smo and SMOM2 decreased the amount of Hhip and HhipΔL2 detected in cell lysates ( Fig. 3a , lanes 3, 5, 13, 15). HhipΔAR, however, was resistant to degradation when co-expressed with Shh, Smo and SMOM2 ( Fig. 3a , lanes 6–10), yet it is an efficient inhibitor of the response in vivo . The EGF domain had no effect on Hhip stability ( Fig. 3b ). Because Smo and Hhip have Frizzled-like CRD domains, we reasoned that CRDs are important interacting domains and therefore may have consequences for Hhip regulation and stability. We tested whether the Smo CRD played a role in the decrease in Hhip protein. Hhip and SmoΔCRD co-transfections did result in an approximately 60% decrease of Hhip compared with over 75% loss of Hhip with Shh, Smo or SMOM2 ( Fig. 3a lane 1–5). This is consistent with the lower activity of SmoΔCRD compared with Smo [19] . HhipΔAR protein was not affected by co-transfection of SmoΔCRD (lane 9). Co-transfection with Ptch1 did not affect Hhip protein in cell lysates ( Fig. 3c , lane 1). Altogether, these results indicate that the instability of Hhip is mediated via its AR domain at the level of or downstream of Smo activation. To further determine whether the activity of the Shh pathway downstream of Smo affects Hhip protein levels, we co-transfected Hhip with the repressor form of Gli3, Gli3R (ref. 20 ; Fig. 3d ). Overexpression of Gli3R did not increase the stability of Hhip, indicating that transcriptional activation of Shh pathway is not involved in the instability of Hhip. Shh induces Smo trafficking to the cell surface and the primary cilium, whereas the Shh/Ptch1 complex traffics to late endosomes [21] , [22] , [23] . As both Shh and Smo dramatically reduce Hhip levels in cells, we assessed if Shh activation results in Hhip internalization and trafficking towards late endosomes and lysosomes for degradation, analogous to Ptch1. Both chloroquine and folimycin A prevent endosome acidification and thus late endosome maturation. Both drugs increased the levels of Hhip and Ptch1 ( Fig. 3d lanes 1–4), indicating that, like Ptch1, the degradation of Hhip occurs in lysosomes. This idea was further supported by the finding that treatment with MG132, a proteasome inhibitor, did not affect Hhip. When Hhip and Shh were coexpressed and treated with these inhibitors, there was a partial rescue of Hhip protein by chloroquine and folimycin A treatment from the Shh-mediated degradation (lanes 5–9). Taken together, these data indicate that both Shh and Smo can induce a rapid internalization of Hhip to degrade it. To further demonstrate that Shh pathway activation increases the turnover of Hhip, we examined the Hhip expression in Ptch1 –/– mouse embryonic fibroblasts (MEFs). In these cells, pathway activity is high because of the absence of Ptch1-mediated inhibition of Smo. Hhip could not be detected in these cells when co-transfected with vector or ShhC ( Fig. 3e ). In contrast, restoring Smo regulation by the co-expression of Ptch1 increased Hhip levels such that it was detectable in this steady-state situation. Chloroquine treatment rescued Hhip in control, ShhC and Ptch1 co-transfected cells, although we could not rescue the effect of Shh on Hhip stability. These data demonstrate that an activated Shh pathway causes lysosomal Hhip degradation. In response to Shh, Hhip has been shown to co-localize with Smo, mediating the internalization of both components [14] . We tested whether stabilization of Hhip protein by mutation or drugs would allow the detection of an interaction between Hhip and Smo. Only upon treatment with chloroquine, Hhip and Smo co-immunoprecipitate, whereas Hhip and SmoΔCRD, co-immunoprecipitated regardless of drug treatment ( Fig. 3f lanes 1–5). HhipΔAR and Smo co-immunoprecipitated with or without chloroquine, yet we detected weak interaction between HhipΔAR and SmoΔCRD (lanes 6–10). These results indicate that both the Hhip AR and the CRD of Smo are not required for interaction, and that the observed interaction was most likely due to the lower activity of SmoΔCRD and the higher stability of HhipΔAR. Activity of Hhip despite cell autonomous Smo activation To determine whether Hhip can still function as an inhibitor of Shh activity when expressed with a Shh activator, we co-electroporated Hhip mutants with SMOM2 or SmoΔCRD in the neural tube. Hb9 was repressed and there was ventral expansion of Pax7 in cells adjacent to those electroporated with Hhip, HhipΔC22 or HhipΔAR and SMOM2, and Hhip and SmoΔCRD ( Fig. 4a–h ). This demonstrates that Hhip non-cell autonomously inhibited the Shh response in nearby cells. SMOM2 and SmoΔCRD effects were strictly cell autonomous because Hb9 expression and Pax7 repression were only observed in Smo electroporated cells. These results also indicate that Hhip did not antagonize the effects of SMOM2 and SmoΔCRD, consistent with the idea that Hhip acts upstream of Smo. But how do these data reconcile with the biochemistry, where SMOM2 expression leads to Hhip degradation? One explanation might be the higher expression levels obtained with electroporation resulting in sufficient release of Hhip to inhibit the Shh response non-cell autonomously. Alternatively, Hhip might be able to bind to Shh that is present in the neural tube before being degraded. 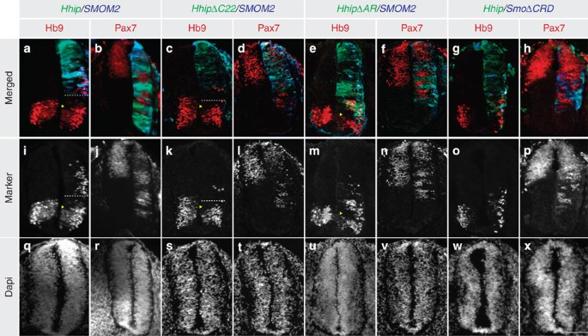Figure 4: Hhip inhibits Shh activity when expressed with a Shh activator. (a–x) Cross-sections of chick neural tubes at stage 20HH. Co-electroporation ofpMES-HhipandpMES-tdTomato-SMOM2(a,b,i,j,q,r),pMES-HA-HhipΔC22andpMES-tdTomato-SMOM2(c,d,k,l,s,t),pMES-HA-HhipΔARandpMES-tdTomato-SMOM2(e,f,m,n,u,v), andpMES-HhipandpMES-tdTomato-SmoΔCRD(g,h,o,p,w,x). Hhip electroporated cells are labelled in green and Smo electroporated cells are labelled in blue. The sections are stained with antibodies to Hb9 or Pax7 and are labelled in red or represented as a grey scale image. (a,i,c,k) The dotted lines mark the boundary of Hhip- and HhipΔC22-expressing cells. Hhip and HhipΔC22 inhibits Hb9 non-cell autonomously as indicated by the yellow arrowheads. The corresponding 4,6-diamidino-2-phenylindole (DAPI) nuclei stain (q–x) to the images above. Scale bar, 50 μm (x). Figure 4: Hhip inhibits Shh activity when expressed with a Shh activator. ( a – x ) Cross-sections of chick neural tubes at stage 20HH. Co-electroporation of pMES-Hhip and pMES-tdTomato-SMOM2 ( a , b , i , j , q , r ), pMES-HA-HhipΔC22 and pMES-tdTomato-SMOM2 ( c , d , k , l , s , t ), pMES-HA-HhipΔAR and pMES-tdTomato-SMOM2 ( e , f , m , n , u , v ), and pMES-Hhip and pMES-tdTomato-SmoΔCRD ( g , h , o , p , w , x ). Hhip electroporated cells are labelled in green and Smo electroporated cells are labelled in blue. The sections are stained with antibodies to Hb9 or Pax7 and are labelled in red or represented as a grey scale image. ( a , i , c , k ) The dotted lines mark the boundary of Hhip- and HhipΔC22-expressing cells. Hhip and HhipΔC22 inhibits Hb9 non-cell autonomously as indicated by the yellow arrowheads. The corresponding 4,6-diamidino-2-phenylindole (DAPI) nuclei stain ( q – x ) to the images above. Scale bar, 50 μm ( x ). Full size image As Hhip inhibited Hb9 in the ventral neural tube even when Hhip electroporated cells were located dorsal to the Hb9 domain and distal to the Shh source ( Fig. 4a ), we examined the consequences of expressing untethered Hhip (HhipΔC22) in the neural tube. Similar to wild-type Hhip, HhipΔC22 inhibited the ventral Hb9 expression when the electroporated cells were located dorsal to the Hb9 domain, demonstrating that both act multiple cell diameters away from the site of synthesis ( Fig. 4c,d ). To assess the functionality of an obligatory membrane-associated form of Hhip, we fused the transmembrane domain and intracellular tail of CD4 to the C-terminal end of HhipΔC22, Hhip:CD4. Robust expression of Hhip:CD4 next to the floor plate and source of Shh repressed Hb9 and deformed the neural tube similar to wild-type Hhip ( Figs 1a and 5a ). Hhip:CD4 induction of Pax7 was completely cell autonomous ( Fig. 5b ). In addition, coexpressing Hhip:CD4 and SMOM2 only resulted in minor non-cell autonomous inhibition of the Shh response ( Fig. 5c,d ). Furthermore, Hhip:CD4 was still susceptible to Shh/Smo-mediated degradation ( Fig. 5m ). These results further indicate that Hhip released from cells mediate part of the non-cell autonomous inhibition. 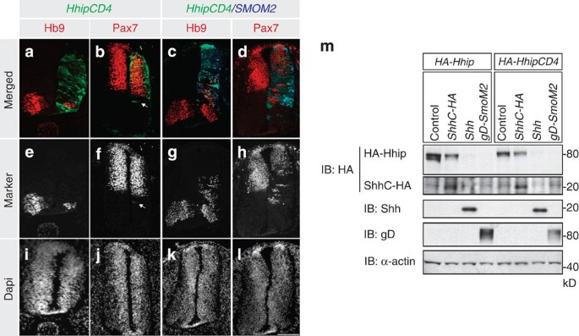Figure 5: Cell tethered Hhip is not as efficient in inhibiting Shh non-cell autonomously as wild type. Chick neural tubes were electroporated withpMES-HA-Hhip:CD4(a,b,e,f,i,j),pMES-HA-Hhip:CD4andpMES-tdTomato-SMOM2(c,d,g,h,k,l). HHip:CD4-expressing cells are labelled in green, SmoM2 cells are labelled in blue and HB9 and Pax7 are labelled in red (a–d). Grey scale images of Hb9 and Pax7 (e–h) and corresponding nuclear 4,6-diamidino-2-phenylindole (DAPI) stain (i–l). Arrow inbandfindicates that Hhip:CD4 inhibition of Pax7 is cell autonomous. Scale bar, 50 μm (l). (m) HEK293T cells were co-transfected withHhip:CD4andShhC,ShhorSmoM2, and Hhip:CD4 was assessed by western blot analysis. Figure 5: Cell tethered Hhip is not as efficient in inhibiting Shh non-cell autonomously as wild type. Chick neural tubes were electroporated with pMES-HA-Hhip:CD4 ( a , b , e , f , i , j ), pMES-HA-Hhip:CD4 and pMES-tdTomato-SMOM2 ( c , d , g , h , k , l ). HHip:CD4-expressing cells are labelled in green, SmoM2 cells are labelled in blue and HB9 and Pax7 are labelled in red ( a – d ). Grey scale images of Hb9 and Pax7 ( e – h ) and corresponding nuclear 4,6-diamidino-2-phenylindole (DAPI) stain ( i – l ). Arrow in b and f indicates that Hhip:CD4 inhibition of Pax7 is cell autonomous. Scale bar, 50 μm ( l ). ( m ) HEK293T cells were co-transfected with Hhip:CD4 and ShhC , Shh or SmoM2 , and Hhip:CD4 was assessed by western blot analysis. Full size image The data shown provide a mechanism by which Hhip is able to act despite being near the Shh source, where Shh can activate the response by enhancing degradation of Hhip, while Hhip retains its non-cell autonomous effects on the Shh response. This explains an inconsistency in the prevailing model in which both Ptch1 and Hhip act as a cell autonomous Shh barrier. The Shh gradient should experience a steep decline in ligand concentrations at the sites of Ptch1/2 and Hhip expression in the neural tube, but such a steep decline of the Shh gradient is not observed. Our data now suggest a graded model where Hhip binds to Shh, both at the cell surface and upon Hhip release from cells, to inhibit the Shh response non-cell autonomously. Consistent with earlier findings, we find that Hhip inhibits the Shh response in neighbouring cells. However, rather than just acting to cell autonomously sequester Shh to lower the amount of Shh available to neighbouring cells, we find that Hhip is also released from the sites of synthesis to inhibit the Shh response at a distance. In particular, our finding that Hhip can inhibit the Shh response in cells that are located between the Shh source and the sites of Hhip synthesis strongly indicates that Hhip is able to act at a distance. Our observation that SmoM2 rescues cells from the consequences of ectopically expressed Hhip from its inhibitory effects raised the question of why the normal sites of Hhip expression have an apparently unimpaired response to Shh. We showed that Shh, Smo or SmoM2 causes a significant loss of cell-associated Hhip, which would counteract the cell autonomous inhibitory activity of Hhip. These results provide a new mechanism by which Hhip is able to act despite being near the Shh source where Shh can activate the response, whereas Hhip retains its non-cell autonomous effects on the Shh response. Besides its signalling functions, Ptch1 plays an important role as negative regulator in shaping the Shh gradient in the neural tube. Hh signalling induces the expression of Ptch1, which leads to more sequestration of Hh ligands, resulting in the creation of a barrier to further movement in the gradient [24] . It was proposed that Hhip functions in a comparable manner [6] . Ptch1 and Hhip expression levels are highest closest to the Shh source. A consequence of the current model, in which both Ptch1 and Hhip act as a cell autonomous Shh barrier, is that the Shh gradient would experience a very steep decline in ligand concentrations at the ventral sites of Ptch1 and Hhip expression in the neural tube. This would most likely cause a pronounced reduction in the expression of ventral progenitors at the induced source of Hhip and Ptch1. Such a steep decline of the Shh gradient is not seen and this prompted us to further examine the role of Hhip regulation of Shh signalling. Our data show a sharp decrease in Hhip when co-expressed with SmoM2, yet, in vivo when Hhip and SmoM2 are co-expressed there remains a robust Hhip non-cell autonomous inhibition of Shh activity. There are several explanations for this discrepancy. First, although there is a drastic decrease in Hhip expression, the remaining Hhip may be enough to inhibit Shh activity. Second, Hhip may have already bound Shh before being degraded. Alternatively, Hhip maintains the ability to inhibit Shh in vivo , because feedback mechanisms are in place where endogenous Hhip and Ptch1 are upregulated by the activated Shh response. This could explain the decrease in Hhip protein expression observed in vitro . Our data provide further evidence of a direct relationship between Hhip and Smo. In zebrafish, Hhip regulates Smo localization, where Smo co-localizes with Hhip at the cell surface, and are internalized together, resulting in Shh pathway inhibition [14] . Although our data are consistent with those previously reported in placing Hhip inhibition of Shh activity upstream of Smo activation [6] , [14] , our study does not address whether Hhip inhibits Shh activity via Smo. Instead, our results indicate that Smo activity regulates Hhip protein levels, even in the absence of Shh binding. Recently, Shh signalling has been implicated in regulating autophagy. In one study, Smo activity downregulated autophagosome synthesis [25] . More recently, Pampliega et al . have shown that Smo regulates cilia-mediated autophaphy [26] . Our result that Smo and Hhip associates in the presence of cholorquine is mostly likely explained by the recent findings that Smo activity is required for Shh-mediated autophagy via ciliogenesis. One important consideration when interpreting our results and comparing them to previously published data is the possibility of overexpressing artefacts. We were unable to detect endogenous Hhip in the tissues studied, and as a consequence, we resorted to introducing Hhip by transfection or electroporation. This allowed us to perform the biochemical and in vivo analyses shown, but could possibly drive Hhip protein to levels that result in perturbed localization of Hhip. However, the ability of specific mutations (ΔARG) to counteract the effects of Smo on Hhip argues against such artefacts. An important consequence of this potential discrepancy between our system and the function and regulation of endogenous Hhip is the interpretation of the causal relationship between the translational induction of Hhip by Smo activation, which is well known, versus the direct action of Smo on Hhip leading to its degradation that we observe. The CRD in the extracellular domain of Smo has been shown to be important in Smo dimerization with implications for Smo activation [27] . In addition, SmoΔCRD has been shown to only mediate low to medium, but not high, levels of pathway activation despite being localized to cilia [19] . The level of Shh pathway activity mediated by Smo determines the fate of Hhip proteins, where high Shh activity decreases Hhip levels most. This is most likely the reason why the Shh response is not impaired where Shh is highly active and where Hhip is most highly expressed. This would also allow Hhip to reduce Shh ligands, as well as alter the localization of Smo, which may decrease the magnitude and duration of the response in various ways. In addition to being targeted by different inhibitory proteins, the stability of Shh ligands also affects how the gradient is maintained. For example, when Ptch1 and Shh bind, the complex is internalized and degraded by the cell, thus rapidly decreasing Shh levels [28] . In contrast, Hhip and Shh complexes appear to be more stable and stay at the cell surface much longer than Ptch1-Shh complexes [6] . With the addition of Hhip being secreted and able to bind to Shh, this adds a new dimension to Hhip’s role in Shh gradient formation. Can Hhip function in a similar manner to other CRD-containing proteins that bind to morphogens to regulate either their activity or range? Examples of these proteins include such molecules as Chordin and soluble Frizzled-related proteins (SFRPs) that bind bone morphogenetic proteins (BMPs) and WNTs/FZDs, respectively. These proteins were both initially thought to inhibit pathway activation, however, data now point to a more complex function for these proteins. For example, SFRP and WNT complexes have been shown to increase long-range WNT signalling [29] . In addition, Chordin binds to BMPs, preventing them from binding their receptors, thus inhibiting activation [30] . However, as Chordin and BMP complexes diffuse in a field, Chordin is cleaved by Tolloid, where this cleavage releases BMP and is allowed to activate the pathway [31] . With all these similarities between Hhip and SFRP and Chordin, it would be interesting to see if Hhip also plays a role in the long-range transport of Shh ligands. Future studies will be needed to address this possibility. Plasmids pcDNA3-mHhip was a gift from Dr P.T. Chuang (University of California, San Francisco). An N-terminal haemagglutinin (HA)-tag was inserted after the Hhip signal sequence following amino-acid 23. Using Quikchange mutagenesis (Agilent Technologies), deletions were created by targeting the following amino acids: 35–54 (HhipΔAR); 373–390 (HhipΔL2); 607–634 (HhipΔEGF) and 669–700 (HhipΔC22). The transmembrane and intracellular domain of CD4 were fused to the C-terminal of HhipΔC22 to make Hhip:CD4. Hhip mutants were also subcloned into pMES-IRES-eGFP or pMES-IRES-tdTomato plasmids for in ovo electroporation. In ovo electroporation Chick embryo electroporation was performed as described [20] . Fertilized White Leghorn chicken eggs (Charles River Laboratories) were incubated at 38 °C until embryos reached Hamburger and Hamilton stage 10. Eggs were windowed, and plasmid DNA resuspended at 2–5 μg μl −1 in PBS was injected into the neural tube of the embryo. Embryos were electroporated between 4 mm gap electrodes at 25 V, 5 × 25 ms pulses with an ECM-820 electroporator (BTX). After electroporation, embryos were incubated until they reached stage 18–20 Hamburger and Hamilton, fixed, incubated in 30% sucrose/PBS overnight, mounted and frozen in OCT compound, and cryosectioned at 12–18 μm. Sections were washed 3 × with PBS/0.01% Triton X-100 and blocked for 30 min with PBS/0.01% Triton X-100 in 5% donkey serum. Sections were immunostained with mouse anti-Pax7 (1:25), mouse anti-Hb9 (1:100) (both from the Developmental Studies Hybridoma Bank) and rabbit anti- green fluorescent protein (GFP; 1:1,000) (Invitrogen) for 2 h at room temperature or overnight at 4 °C. After washing with PBS/0.01% Triton X-100, the appropriate secondary antibodies added and were incubated for 1 h. Images were obtained using routine fluorescence microscopy techniques on a Microphot-SA epifluorescence microscope (Nikon) or an Axio Observer Z1 (Zeiss) fluorescence microscope. Immunofluorescent staining Madin–Darby canine kidney cells (ATCC, CCL-34) were transfected with either pcDNA3.1-HA-Hhip, including a plasmid expressing GFP, or pRK5-Shh using Lipofectamine LTX and Plus Reagent (Invitrogen). After 24 h, cells were detached, mixed together and cultured overnight. Cells were fixed using 4% formaldehyde in PBS, blocked with PBS/0.01% Triton X-100 with 5% goat serum and subsequently incubated with the following primary antibodies: rat anti-HA (1:500; 3F10, Roche Applied Science) and rabbit anti-Shh (1:100; H160, SCBT) overnight at 4 °C. Slides were washed and then incubated with the following secondary antibodies: Alexa-488 anti-Rat IgG and Alexa-568 anti-rabbit (1:1,000; Invitrogen). Cell images were acquired on an Axio Observer Z1 microscope. Co-immunoprecipitation and co-expression HEK 293T cells (ATCC, CRL-3216) were transfected with DNA using Lipofectamine 2000 (Invitrogen). For co-immunoprecipitation, cells were detached with PBS/0.5 mM EDTA 24 h after transfection, and co-cultured overnight in Optimem (Invitrogen). Supernatants were collected and cleared by centrifugation. Cells were lysed (25 mM HEPES, 150 mM NaCl, 1% IGEPAL CA-630, 1 mM Na 3 VO 4 and protease cocktail inhibitor) and cleared. Lysates and supernatants were immunoprecipitated with Hhip antibody (1.6 μg per sample; M-17, SCBT) or anti-HA (4 μl per sample; Sigma). For co-expression experiments, HEK 293T cells were co-transfected as for the co-culture experiments. For the inhibition of degradation, cells were treated with chloroquine (Sigma), folimycin A (Calbiochem) or MG132 (Calbiochem). After 48 h, cells were directly lysed in 1 × NuPAGE LDS sample buffer (Invitrogen). Lysates were run on NuPAGE precast gels (Invitrogen) and transferred to membrane using the iBlot gel transfer system. Membranes were blocked in 5% milk in TBS/0.1% Tween-20 for 1 h and incubated in the following primary antibodies overnight at 4 °C: rat anti-HA (1:10,000); rabbit anti-Shh (1:1,000) antibody, mouse-anti-myc (1:10,000; 9B11, Cell Signaling Technology) and mouse anti-gD (1:10,000; clone ID3). The next day, membranes were washed and incubated in the appropriate secondary antibodies (1:10,000) for 1–3 h and enhanced chemiluminescence (ECL) was imaged using film. Uncropped images of HA and Hhip blots are shown in Supplementary Fig. 1 . Conditioned Hhip and ShhN medium and luciferase assays HEK 293T cells were transfected using Lipofectamine 2000 with empty vector control, Hhip mutants or ShhN DNA. One day after transfection, cells were washed with PBS and the medium was switched to Optimem. After another 48 h, cell medium was collected and used in the co-culture assay. For the co-culture assay, MIA PaCa-2 cells (ATCC CRL-1420) were cultured together with Shh-LIGHT II cells (ATCC CRL-2795) at 10 6 cells in 5 ml DMEM containing 0.5% FCS in 60 mm dishes on rotary shaker at 55 r.p.m. After spheroid cultures formed (typically 3d), Hhip conditioned medium or 5E1 antibody was added for an additional 24 h. Cells were lysed and Gli-luciferase activity was assayed using the Dual Luciferase Reporter Assay Kit (Promega). Relative luminescence units were measured on a Victor plate reader (Perkin Elmer) and corrected for an internal cytomegalovirus-driven Renilla luciferase control. How to cite this article : Kwong, L. et al . Shh-mediated degradation of Hhip allows cell autonomous and non-cell autonomous Shh signalling. Nat. Commun. 5:4849 doi: 10.1038/ncomms5849 (2014).